The formation of unsaturated IrOxin SrIrO3by cobalt-doping for acidic oxygen evolution reaction Electrocatalytic water splitting is a promising route for sustainable hydrogen production. However, the high overpotential of the anodic oxygen evolution reaction poses significant challenge. SrIrO 3 -based perovskite-type catalysts have shown great potential for acidic oxygen evolution reaction, but the origins of their high activity are still unclear. Herein, we develop a Co-doped SrIrO 3 system to enhance oxygen evolution reaction activity and elucidate the origin of catalytic activity. In situ experiments reveal Co activates surface lattice oxygen, rapidly exposing IrO x active sites, while bulk Co doping optimizes the adsorbate binding energy of IrO x . The Co-doped SrIrO 3 demonstrates high oxygen evolution reaction electrocatalytic activity, markedly surpassing the commercial IrO 2 catalysts in both conventional electrolyzer and proton exchange membrane water electrolyzer. Water splitting for hydrogen production offers the advantage of producing clean and sustainable fuel without carbon emissions [1] , [2] . To date, proton exchange membrane (PEM) water electrolysis is one of the most established ways in the field of green hydrogen production [3] , [4] , [5] . However, the high overpotential typically associated with the anodic oxygen evolution reaction (OER) poses a significant challenge to enhancing hydrogen production efficiency from water electrolysis [6] . Furthermore, the advancement of OER catalysts designed for acidic medium poses a greater challenge compared to those intended for alkaline medium. Since highly OER-active electrocatalysts are mainly comprised of metal oxides or hydroxides, most of which exhibit poor stability under acidic conditions [7] , [8] , [9] , [10] . Therefore, the development of efficient OER catalysts functioning in acidic medium is critical. Current, effective acidic OER catalysts include Ru, Ir, and Mn-based metal oxides [11] , [12] , [13] , [14] , [15] , [16] , [17] . In particular, SrIrO 3 with an ABO 3 perovskite structure (where A typically represents an alkaline earth metal and B represents a transition metal) shows high acidic OER catalytic performance [18] , [19] , [20] , [21] , [22] , [23] , [24] , [25] , [26] , [27] , [28] , [29] , [30] . In recent years, extensive researchers have been conducted to understand the OER catalytic mechanism of SrIrO 3 . Jaramillo et al. prepared the (001) plane SrIrO 3 film via a laser epitaxy strategy, and observed an incremental improvement in its OER catalytic performance throughout the catalytic process [22] . Through combining theoretical calculations and experiments, they discovered that the high catalytic activity of SrIrO 3 could be attributed to the exposed IrO x sites following Sr dissolution. In further comprehensive studies, researchers confirmed the structural modifications of SrIrO 3 under acidic OER process using secondary ion mass spectrometry (SIMS), in situ atomic force microscopy (AFM), and X-ray absorption spectroscopy (XAS), respectively [23] , [24] , [25] . They proposed a correlation between the Sr dissolution process and the formed IrO x surface activities. Moreover, an investigation involving SrIr 0.1 Co 0.9 O 3 further indicates that the OER activity also originates from the amorphous IrO x structure formed by the dissolution of Co [26] . These studies appear to identify the active component of SrIrO 3 -based perovskites as the amorphous IrO x structure. Nevertheless, most studies overlook the impact of B-site dissolution on surface oxygen stability and Ir-O coordination structure, the precise reasons contributing to the high OER catalytic performance of Co-doped SrIrO 3 catalysts remain unclear. This issue primarily stems from the challenge faced by researchers in elucidating two key aspects of the OER catalytic process: (1) The key role of Co dissolution in catalytic processes and (2) the influence of surface and bulk Co on IrO x sites. To address the two key challenges mentioned above, we designed a B-site Co-doped SrIrO 3 system to discern the dissolution mechanism at catalyst sites and the origins of IrO x catalytic activity, as shown in Fig. 1a . In situ inductively coupled plasma mass spectrometry (ICP-MS) experiments revealed simultaneous ion dissolution of Co and Sr, caused by acid corrosion prior to OER process. At the OER potential (1.60 V vs. RHE), the dissolution phenomenon was found to be negligible. Along with theoretical calculations, a series of in situ experiments including in situ Raman mapping, in situ XAS, and differential electrochemical mass spectrometry (DEMS) were conducted. These results highlighted the role of Co in two critical ways: (1) Surface Co reduces the stability of the Co-O-Ir bridge oxygen in SrIrO 3 , leading to the rapid exposure of the low-coordination IrO x structure; (2) Bulk lattice Co optimizes the OOH binding energy of IrO x , consequently reducing the overpotential. Thus, the synthesized Co-doped SrIrO 3 demonstrated high OER activity, markedly surpassing commercial IrO 2 catalysts in PEM water electrolyzer. The insights obtained from this research would significantly enhance the understanding of high OER catalytic performance of SrIrO 3 -based perovskite catalysts, providing key insights for designing and preparing high-performance acidic OER catalysts. Fig. 1: Characterizations of samples. a OER catalytic mechanism diagram of Co-doped SrIrO 3 catalyst; b – d HRTEM images and corresponding FFT diagrams of SI, SI 6 C 1 and SI 1 C 1 ; e O K -edge EELS spectra of SI 6 C 1 ; f HAADF image of SI 6 C 1 and corresponding EDS mapping images; g , h XRD spectra of SI 1 C 1 , SI 2 C 1 , SI 4 C 1 , SI 6 C 1 , SI 8 C 1 , and SI samples. i ICP–MS diagram of Co/Ir and Sr/Ir ratios of SI 1 C 1 , SI 2 C 1 , SI 4 C 1 , SI 6 C 1 , SI 8 C 1 , and SI samples. Full size image Fabrication and characterizations of Co-doped SrIrO 3 samples SrIrO 3 doped with different amounts of Co were synthesized by using the sol-gel method, and were fully acid washed before use. The samples were denoted as follows: Sr 2 IrCoO x (SI 1 C 1 ), Sr 3 Ir 2 CoO x (SI 2 C 1 ), Sr 5 Ir 4 CoO x (SI 4 C 1 ), Sr 7 Ir 6 CoO x (SI 6 C 1 ), Sr 9 Ir 8 CoO x (SI 8 C 1 ), and SrIrO x (SI). The crystal structures of these samples were analyzed through high-resolution transmission electron microscopy (HRTEM) and X-ray diffraction (XRD) in Fig. 1 b– h , respectively. For HRTEM testing, three samples (SI, SI 6 C 1 , and SI 1 C 1 ) were selected. Specifically, SI exhibited an orthorhombic crystal structure. Fast Fourier transform (FFT) showed that the primary exposed crystal planes included (112), (110), and (002). Despite its low surface crystallinity, SI 6 C 1 still clearly exposed crystal planes such as (112), (204), and (020). Meanwhile, SI 1 C 1 displayed poor surface crystallinity with only a few areas showing short-range ordered crystallinity and no clear diffraction spots in the FFT pattern. To investigate the reason for the diminished crystallinity observed in SI 6 C 1 sample, we conducted electron energy loss spectroscopy (EELS) analyses, the results of which are presented in Fig. 1e and Supplementary Fig. 3 . The peaks at 532, 542, and 564 eV can be ascribed to the Ir 5d, while the peak at 536 eV is attributable to the Sr 4d [31] , [32] . Comparative analysis reveals that the Sr 4d peak of the SI sample is generally higher than that of the SI 6 C 1 sample, suggesting that the presence of Sr contributes to maintaining the crystalline structure. Moreover, we identified a significant discrepancy between the surface and bulk Sr concentrations within the SI and SI 6 C 1 samples, with this effect being particularly pronounced in the SI 6 C 1 sample. This indicates that Co dissolution also impacts the proportion of Sr presenting on the surface. Further investigations were undertaken through energy-dispersive X-ray spectroscopy (EDS) mapping (Fig. 1f ). The results confirm that the dissolution of Sr/Co and the subsequent formation of IrO x . XRD revealed that the diffraction peaks of SI were consistent with typical pseudocubic (Pnma) perovskites. Also, Co-doped SI also demonstrated similar diffraction peaks, confirming the successful synthesis of the perovskite-based catalyst [21] , [26] . As shown in Fig. 1h , Co doping significantly reduced the crystallinity of SI and resulted in the diffraction peak shifting to the high angle, indicating lattice contraction in the Co-doped SI. In particular, SI 1 C 1 and SI 2 C 1 displayed almost no diffraction peaks, possibly due to the substantial dissolution of surface Co and Sr by acid washing process. These findings suggest that excessive Co doping may disrupt the pseudocubic perovskite structure after acid washing, a conclusion in line with the HRTEM results. The overall composition of the samples was analyzed by using ICP-MS, as shown in Fig. 1i . Notably, there was a significant discrepancy between the Co and Ir initial ratio and the final composition ratio of the samples. Samples with poor crystallinity, specifically SI 1 C 1 and SI 2 C 1 , exhibited the highest Co/Ir ratio, with SI 2 C 1 slightly higher than SI 1 C 1 . This could possibly be attributed to the difficulty in maintaining the perovskite structure in SI 1 C 1 , which led to a large amount of Co dissolution during the acid washing process and, consequently, a reduced Co/Ir ratio. Despite possessing the highest Co/Ir ratios, these two samples were still significantly lower than the initial ratio, further confirming the instability of surface Co in acidic conditions. The Co/Ir ratios of SI 4 C 1 , SI 6 C 1 , and SI 8 C 1 showed a decreasing trend from SI 4 C 1 , SI 6 C 1 to SI 8 C 1 as shown in. 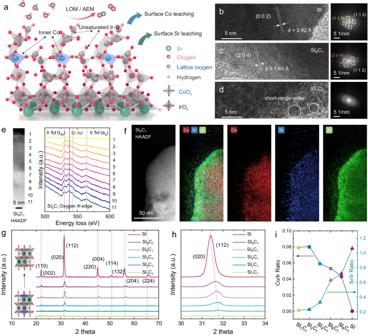Fig. 1: Characterizations of samples. aOER catalytic mechanism diagram of Co-doped SrIrO3catalyst;b–dHRTEM images and corresponding FFT diagrams of SI, SI6C1and SI1C1;eOK-edge EELS spectra of SI6C1;fHAADF image of SI6C1and corresponding EDS mapping images;g,hXRD spectra of SI1C1, SI2C1, SI4C1, SI6C1, SI8C1, and SI samples.iICP–MS diagram of Co/Ir and Sr/Ir ratios of SI1C1, SI2C1, SI4C1, SI6C1, SI8C1, and SI samples. Figure 1i suggesting that lattice maintenance assists in stabilizing Co atoms in the bulk phase. Among various SI-based samples, the SI 1 C 1 and SI 2 C 1 displayed the lowest Sr/Ir ratio, and the Sr/Ir ratio significantly increased with the decrease of Co doping. The Sr/Ir ratio of the SI sample was slightly higher than 1, indicating a slightly higher Sr proportion compared to Ir in bulk structure, as suggested by the EELS results shown in Supplementary Fig. 3 . These conclusions were further confirmed by additional characterization methods such as scanning electron microscope (SEM), X-ray photoelectron spectroscopy (XPS), and Raman spectroscopy, as shown in Supplementary Fig. 5a, b . High OER catalytic performance of Co-doped SrIrO 3 The OER catalytic performances of the SI 1 C 1 , SI 2 C 1 , SI 4 C 1 , SI 6 C 1 , SI 8 C 1 , and SI samples were investigated in acidic medium. The linear sweep voltammetry (LSV) curves for SI 1 C 1 , SI 2 C 1 , SI 4 C 1 , SI 6 C 1 , SI 8 C 1 , and SI samples were recorded after 10 cyclic voltammetry (CV) cycles, as shown in Fig. 2a . The results indicate that SI 6 C 1 necessitates an overpotential of only 245 mV to reach a current density of 10 mA/cm 2 , which is approximately 5 times higher than that of SI at the same potential. Given that the OER catalytic process primarily occurs on the surface, the performance of SI 1 C 1 , SI 2 C 1 , SI 4 C 1 , SI 6 C 1 and SI 8 C 1 samples is generally superior and exhibits a similar trend. This aligns with previous characterization results, suggesting that despite varying Co doping ratios, the catalysts’ surface structures are comparable. As presented in Fig. 2b, c , the SI 1 C 1 , SI 2 C 1 , SI 4 C 1 , SI 6 C 1 and SI 8 C 1 samples show Tafel slopes within the range 51.5–53.6 mV/dec, significantly lower than that of SI (59.5 mV/dec). This suggests that Co participation can enhance the reaction kinetics of OER. As shown in Fig. 2 d, a comparison of the mass activity of the SI 1 C 1 , SI 2 C 1 , SI 4 C 1 , SI 6 C 1 , SI 8 C 1 , SI and IrO 2 samples reveals that the Co-doped samples all demonstrated high activity, significantly surpassing those of SI and IrO 2 . Fig. 2: Electrochemical measurements of samples. a OER polarization curves of SI 1 C 1 , SI 2 C 1 , SI 4 C 1 , SI 6 C 1 , SI 8 C 1 , and SI samples with a mass loading of 0.025 mg/cm 2 in 0.5 M H 2 SO 4 and ( b ) corresponding Tafel slopes. The resistance values for SI 1 C 1 , SI 2 C 1 , SI 4 C 1 , SI 6 C 1 , SI 8 C 1 , SI and IrO 2 were 3.9, 3.7, 3.6, 4.7, 3.2, 4.6 and 4.4 Ω, respectively. c Comparison of overvoltages and Tafel slopes of SI 1 C 1 , SI 2 C 1 , SI 4 C 1 , SI 6 C 1 , SI 8 C 1 , and SI samples. d Comparison of OER mass activity of SI 1 C 1 , SI 2 C 1 , SI 4 C 1 , SI 6 C 1 , SI 8 C 1 , SI and IrO 2 samples. e Schematic diagram of PEM water electrolysis device. f PEM water electrolysis performance of SI 6 C 1 , IrO 2 , and SI samples, in set: PEM water electrolysis device photograph. g PEM water electrolysis stability of SI 6 C 1 sample. Full size image To study the potential applications of SI series catalysts in water electrolysis, we further examined the electrocatalytic performance of three samples (SI, SI 6 C 1 , and IrO 2 ) for water electrolysis by PEM. The schematic diagram of the PEM water electrolyzer is presented in Fig. 2e . The performance results of the PEM water electrolysis, shown in Fig. 2f , reveal that the catalytic activity of SI 6 C 1 is significantly higher than those of SI and IrO 2 . It can achieve a current density exceeding 1000 mA/cm 2 at 2.0 V cell voltage at 85 °C, which is much higher than those of the SI catalyst (580 mA/cm 2 ) and IrO 2 catalyst (560 mA/cm 2 ) under the same conditions. We further tested the long-term stability of SI 6 C 1 catalyst for PEM water electrolysis as shown in Fig. 2g and Supplementary Fig. 6 . The results indicate that the SI 6 C 1 catalyst exhibits high stability, with a performance decay rate of 0.21 mV/h, which is comparable to that of the SI catalyst and commercial IrO 2 catalyst. This exceptional high stability indicates that the SI 6 C 1 catalyst exhibits the potential for practical application in PEM water electrolysis. The roles of Co doping and dissolution in SrIrO 3 studied by theoretical calculations The impact of Co doping on SrIrO 3 was investigated through a theoretical study. As numerous early studies had substantiated that SrIrO 3 -based catalysts undergo significant Sr dissolution during OER [23] , [24] , [25] . This was examined by analyzing the Pourbaix diagrams of SrIrO 3 and Sr 4 Ir 3 CoO 12 , particularly focusing on their stability in acidic medium (Fig. 3a and Supplementary Fig. 7 ). The findings reveal a marked similarity in the stability properties of SrIrO 3 and Sr 4 Ir 3 CoO 12 . Under acidic conditions, Sr displays a thermodynamic inclination towards dissolution, thereby exposing a multitude of IrO x sites on the surface. Additionally, Co in the Sr 4 Ir 3 CoO 12 also exhibits instability in acidic medium, which could also result in substantial dissolution, consistent with the EDS mapping and ICP-MS results in Fig. 1 . Fig. 3: Theoretical calculations of SrIrO 3 -based perovskite catalysts. a Pourbaix diagram of SrIrO 3 . b Possible computational models of IrO x , IrCo surf O x (surface Co doping) and Ir unsat Co 2L O x (second layer Co doping with unsaturated IrO x ) for DFT calculations. c Adsorbate evolution mechanism (AEM) diagram. d OER free energy diagrams of different models. e Overpotential of different computational models. f Density of states diagrams for IrO x and Ir unsat Co 2L O x , and ( g , h ) energy band center and volcano plot for different computational models. Full size image As indicated by the Pourbaix diagram, the structure of catalyst is significantly influenced by the applied voltage. However, the two catalysts do not exhibit notable thermodynamic differences near the oxygen stability curve, although they display pronounced differences in thermodynamic tendencies across varying pH values. This suggests that the effect of SrIrO 3 dissolution at different OER potentials may be significantly less than the effect of electrolyte pH, particularly in strongly acidic medium. Previous research suggests that the Ir-O coordination number of surface IrO x on SrIrO 3 during OER catalysis is ~4.5 [25] . While the presence Sr content at the trace amount has been detected in numerous studies, determining the exact state of Sr at the subnanometer scale remains a challenge [23] . By combining the results from the Pourbaix diagrams and above characterizations, seven models were constructed to investigate the theoretical OER catalytic sites and catalytic performance of SrIrO 3 and Co-doped SrIrO 3 (Fig. 3b and Supplementary Fig. 8 ). The theoretical calculations were conducted on the models, as shown in Fig. 3c . The computed free energy diagrams (Fig. 3d ) reveal that the rate-determining step for all models is the formation of *OOH. The Co doping, whether at the surface and bulk phase, which would not change the coordination structure of IrO 6 octahedron, can only enhance OER catalytic activity to a certain extent. However, such activity enhancements are restricted, especially for bulk-doped Co, where the OER overpotential is reduced by only 15 ~ 42 mV. In contrast, the surface unsaturated IrO x , which forms following Co dissolution, exhibits a significant improvement in the catalytic activity for oxygen evolution, with the overpotential decreasing by 311 ~ 344 mV (Fig. 3e ). These findings suggest that Co may not directly participate in the catalysis, but rather promote the surface reconstruction through site dissolution, leading to rapid exposure of more low-coordination IrO x active sites. To further investigate the activity origin, density of states (DOS) analyses were performed on these models (Fig. 3f ). The data suggest that Co doping significantly affects the Co-O-Ir bridge oxygen, shifting the O 2 p band center closer to the Fermi level. According to the related studies, such a shift in the O 2 p band center substantially affect the surface stability of the catalyst and may be associated with oxygen dissolution [33] , [34] . This indicates that the primary effect of Co doping is to alter the surface stability of SrIrO 3 , and promote the surface reconstruction and the formation of IrO x active sites. Additionally, the doping and dissolution of Co significantly influence the Ir 3 d band center (Fig. 3g ). The displacement of the metal 3 d orbitals typically directly impacts the binding energy to the adsorbate. In this study, the negative shift of the Ir 3 d band center led to a decrease in *OOH free energy, significantly enhancing the OER catalytic activity (Fig. 3g ). By establishing the relationship between the Ir 3 d and O 2 p band centers and the theoretical overpotential, a new OER volcano plot was formulated (Fig. 3h ). The data revealed that the moderate O 2 p band center and the lower Ir 3 d band center play crucial roles in the catalytic activity of SrIrO 3 -based catalysts. In situ characterizations of surface structural changes of catalysts To elucidate the catalytic mechanism, DEMS tests were first conducted, as shown in Fig. 4a . The surfaces of SI 1 C 1 , SI 2 C 1 , SI 4 C 1 , SI 6 C 1 , SI 8 C 1 , SI, and IrO 2 samples were labeled with 18 O, as shown in Supplementary Figs. 10 – 12 . For each sample, m / z = 34 signals at different cyclic voltammetry cycles were collected, and the ratio of 18 O 16 O to 16 O 2 was utilized to eliminate the natural abundance of 18 O in the air. As shown in Supplementary Fig. 13 , the lattice oxygen evolution reaction (LOER) trend of most catalysts across different cyclic voltammetry cycles is similar, and the Co doping ratio appears to facilitate the release of lattice oxygen. The results indicated that Co doping reduces the stability of the surface oxygen in SrIrO 3 , consistent with O 2 p center calculation results . Notably, the LOER of SI 1 C 1 and SI 2 C 1 is the most prominent, with SI 2 C 1 slightly surpassing SI 1 C 1 . This phenomenon has been previously explained by XRD and ICP-MS characterizations, as SI 1 C 1 has difficulty in maintaining the perovskite lattice, the proportion of Co doping decreases. In contrast, SI and IrO 2 exhibit the smallest LOER process, which is linked to the stability of the catalyst surface lattice oxygen. The results indicated that Co doping and dissolution can activate the catalyst lattice oxygen, thereby accelerating the formation of IrO x . Fig. 4: In situ characterizations of samples. a The 18 O 16 O percentage of the samples test by DEMS. b In situ ICP-MS diagram of SI and SI 6 C 1 and ( c ) its differential transformation diagram, in set: enlarged diagram. d , e In situ Raman and Raman mapping of SI samples and SI 6 C 1 samples. Full size image In addition to LOER, in situ ICP-MS experiments were performed to detect the phenomenon of ion dissolution during OER, as shown in Fig. 4b, c . We observed that both SI 6 C 1 and SI undergo considerable dissolution when immersed in an acidic electrolyte. Coupling this observation with prior XRD and Raman results, it suggests that the dissolution process is triggered by the rapid dissolution of Sr/Co-related oxides or compound heterophases. Furthermore, the subsequent steady dissolution trend indicates that ion dissolution of the catalyst does not necessarily occur during the catalytic process. It is noteworthy that the Sr dissolution phenomenon of SI is more significant than that of SI 6 C 1 , which is attributed to the higher concentration of surface and bulk Sr in SI. Moreover, SI 6 C 1 is also accompanied by a small amount of Co dissolution, thus further confirming that Co dissolution promotes the formation of unsaturated IrO x . To confirm the structural information of the catalyst, an in situ Raman mapping study was conducted, as shown in Fig. 4d, e . The peak around 600 cm −1 can be attributed to the Ir- μ -oxo stretching vibration of IrO x (involving the unprotonated bridge oxygen, Ir 3+ ), and the characteristic peaks around 550 cm −1 and 720 cm −1 can be attributed to the typical E g and B 2g vibrational peaks of IrO 2 . In addition, the characteristic peaks around 300 and 700 cm −1 can be attributed to Sr-related oxide or compound [35] , [36] , [37] , [38] . The figure shows that before and after the OER process, SI exhibits an obvious Ir- μ -oxo stretching vibration peak at 600 cm −1 , confirming the existence of the perovskite IrO 6 structure. However, for SI 6 C 1 , a significant decrease in the Ir- μ -oxo stretching vibration peak is observed. This may be attributed to the destruction of the IrO 6 structure by Codissolution to form the low-coordination IrO x structure, leading to a significant reduction in peak intensity. Moreover, the characteristic peaks of Sr-related oxides/compounds near 300 and 700 cm −1 nearly disappear from the open circuit voltage (OC). Together with the results of in situ ICP–MS, it can be further confirmed to be caused by the dissolution of Sr-related oxides/compounds. Key evidences of highly active low-coordination IrO x in Co-doped SrIrO 3 for OER To elucidate the formation mechanism of IrO x on the surface, comprehensive in situ EXAFS spectra was recorded at the Ir- L III edge to monitor the evolution of local coordination of Ir, as shown in Fig. 5a–e . Initially, we examined the coordination changes of the SI sample, as demonstrated in Fig. 5a, b . The pristine state SI sample owns a Ir-O coordination number of 5.6, indicating the existence of substantial intact Ir-O octahedral structure within the catalyst. During the pre-OER stage (OC, 1.23 V, 1.43 V vs. RHE), the Ir-O coordination numbers of SI sample exhibited a pattern of initial increase followed by a decrease. Fig. 5: In situ XAS characterization of samples. a R-space fitting diagram for SI sample. b Changes in Ir-O coordination and Ir-O bond length of SI sample. c Structure change diagram of SI sample; d R-space fitting diagram of SI 6 C 1 sample. e Ir-O coordination and Ir-O bond length variation diagram of SI 6 C 1 sample. f Structure change diagram of SI 6 C 1 sample. g Ir– L III Absorption edge diagram of SI sample, in set: enlarged diagram. h Ir– L III absorption edge diagram of SI 6 C 1 sample, in set: enlarged diagram. Full size image Previous reports showed a significant augmentation in the Ir-O coordination number of SrIrO 3 thin film samples during OER, which was ascribed to the oxygen refilling process [24] , [25] . In this study, the dissolution of Sr led to alterations in the surface structure of SI. However, there was no significant LOER in SI sample. Therefore, during the OER oxidation process, the rate of H 2 O filling exceeded the rate of LOER, resulting in the observed trend in coordination numbers. During the OER stage (1.63 V vs. RHE), the Ir-O coordination number of the SI sample exhibited a minor increase, suggesting that at high potentials, the lattice oxygen of SI remained inactive, leading to the higher H 2 O filling rate than the LOER rate [25] . Additionally, at 1.23 V vs. RHE, a significant reduction in the Ir-O bond length of the SI sample was observed, potentially indicating a transformation of the octahedral corner-sharing structure during the H 2 O filling process [26] . In sum, as shown in Fig. 5c , the surface site mechanism of the SI sample undergoes a dynamic process from a relatively complete perovskite structure to site dissolution and adsorbate filling, ultimately transitioning into a saturated IrO x structure. We next analyzed the coordination changes in the SI 6 C 1 sample, as illustrated in Fig. 5d, e . The initial Ir-O coordination number of SI 6 C 1 was 6.0, suggesting a more perfect Ir-O octahedral structure compared with SI. However, prior to the OER stage (OC, 1.23 V, 1.43 V vs. RHE), the Ir-O coordination number of the SI 6 C 1 sample exhibited a notable decreasing trend. This is consistent with the formation of low-coordination IrO x as observed in in situ ICP-MS results. Furthermore, during the OER stage, the Ir-O coordination number of SI 6 C 1 further decreased to 5.4, significantly lower than SI, confirming that the active lattice oxygen in SI 6 C 1 further facilitated the formation of highly active low-coordination IrO x . To validate the generation of the unsaturated IrO x structure, in situ XANES spectra were analyzed at the Ir- L III edge to study the oxidation state of Ir, as shown in Fig. 5g, h . The Ir- L III absorption edge of SI displayed an increasing white line intensity during the OER process, indicating an increase in the oxidation state of Ir. Differently, the Ir- L III absorption edge of SI 6 C 1 exhibited a slight decrease in white line intensity, signifying a reduction in the oxidation state of Ir. Combined with the valence state information of reference samples Ir and IrO 2 , the mechanism of Ir valence state change during OER can be inferred. During the OER process of SI, the dissolution of Sr and the filling of H 2 O led to the saturation of the Ir-O coordination, displaying a higher valence state. Conversely, for SI 6 C 1 , the dissolution of Co resulted in the formation of unsaturated Ir-O, leading to a decrease in the average Ir valence state. This observation further substantiates that Co can enhance the generation of unsaturated IrO x structures, aligning with the results from prior characterizations. OER catalytic mechanism on Co-doped SrIrO 3 catalyst Our study has elucidated the surface reconstruction process of SIC series catalysts by theoretical calculations and a comprehensive series of in situ characterizations. We now proceed to discuss and summarize the potential OER mechanisms inherent to SIC series catalysts. There are two widely recognized mechanisms for OER, specifically the adsorbate evolution mechanism (AEM) and the lattice oxygen mechanism (LOM), as shown in Fig. 6a, b [39] , [40] . 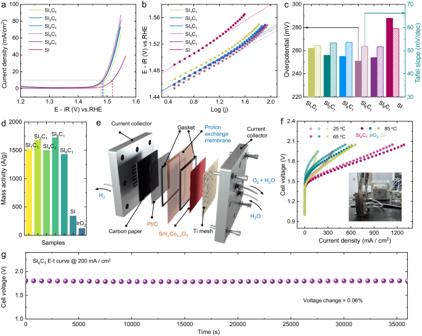Fig. 2: Electrochemical measurements of samples. aOER polarization curves of SI1C1, SI2C1, SI4C1, SI6C1, SI8C1, and SI samples with a mass loading of 0.025 mg/cm2in 0.5 M H2SO4and (b) corresponding Tafel slopes. The resistance values for SI1C1, SI2C1, SI4C1, SI6C1, SI8C1, SI and IrO2were 3.9, 3.7, 3.6, 4.7, 3.2, 4.6 and 4.4 Ω, respectively.cComparison of overvoltages and Tafel slopes of SI1C1, SI2C1, SI4C1, SI6C1, SI8C1, and SI samples.dComparison of OER mass activity of SI1C1, SI2C1, SI4C1, SI6C1, SI8C1, SI and IrO2samples.eSchematic diagram of PEM water electrolysis device.fPEM water electrolysis performance of SI6C1, IrO2, and SI samples, in set: PEM water electrolysis device photograph.gPEM water electrolysis stability of SI6C1sample. Our theoretical calculations have demonstrated that the surface O 2 p band center of the Co/Ir model is closer to the Fermi level compared to the Ir model, which suggests that the bridging oxygen of Co-O-Ir is thermodynamically predisposed to be oxidized [40] . In situ Raman spectroscopy revealed that the Ir- μ -oxo stretching vibration peak (indicative of bridging oxygen) in the Co/Ir system catalyst was notably reduced during the OC and OER processes when compared to the Ir system. Further, DEMS tests have found that a higher content of Co promotes the LOM. Fig. 6: Proposed possible OER mechanism. a Adsorbate evolution mechanism. b Lattice oxygen mechanism. c Lattice oxygen promoted adsorbate evolution mechanism. d Catalytic mechanism of Co-doped SrIrO 3 catalyst. Full size image Despite these findings, our DEMS results suggest that the AEM remains the dominant mechanism, while the LOM significantly contributes to the formation of unsaturated IrO x . Consequently, we propose a distinctive catalytic mechanism, the lattice oxygen promoted adsorbate evolution mechanism (LOPAEM), as illustrated in Fig. 6c . Unlike the conventional catalytic mechanisms of OER, LOPAEM involves the synergistic action of both mechanisms. Specifically, when the oxidation rate of lattice oxygen in certain catalysts becomes excessively fast, it will lead to the formation of a large number of surface oxygen vacancies (i.e., unsaturated metal sites), thereby altering the original catalytic sites of the catalyst. These unsaturated metal sites may exhibit more efficient AEM performance, thus achieving LOPAEM. Our findings suggest that the LOM in Co/Ir system catalysts is an integral step for catalyst activation. The formation of Ir-O-Co vac substantially reduces the catalyst’s AEM overpotential, thereby making it thermodynamically more favorable. This is in agreement with our theoretical calculations and DEMS results. Moreover, the LOM process is unable to produce a lower Ir-O coordination structure as the dissolution of lattice oxygen shifts the O 2 p center away from the Fermi level, precluding further oxidation (as detailed in the theoretical calculation section). In light of the above findings, we have summarized the mechanism for the Co/Ir system catalyst as represented in Fig. 6d . Initially, Co on the catalyst’s surface dissolves under acidic conditions, removing a portion of the bridging lattice oxygen to form an IrO x structure with lower coordination. Subsequently, lattice oxygen dissolves during the OER process, forming an unsaturated IrO x structure that exhibits high AEM activity. Lastly, under the dynamic balance of adsorbate filling and LOM, the catalyst conducts AEM to efficiently facilitate the OER. In summary, we designed a highly active catalyst through Co doping and dynamic dissolution of Co/Sr bimetallic ions to study the catalytic mechanism of SrIrO 3 -based perovskite. Theoretical calculations and in situ characterizations (DEMS, in situ Raman mapping, in situ XAS and in situ ICP-MS) show that dynamic dissolution of Co is crucial for forming highly active unsaturated IrO x . The as-synthesized catalysts exhibit higher OER reaction kinetics than SrIrO 3 and commercial IrO 2 catalyst in both electrolyzer and PEM water electrolyzer, revealing the mechanism of catalytic activity enhancement by tuning catalytic sites. This work is of great significance for understanding the high OER catalytic performance of Ir-based catalysts, and will provide an important basis for the design and preparation of high-performance acidic OER catalysts. Chemicals The chemical reagents utilized in this study were all received from the manufacturer. Potassium hexachloroiridate (IV) [K 2 IrCl 6 , AR, Macklin], cobalt(III) nitrate hexahydrate [Co(NO 3 ) 3 ·6H 2 O, AR, Sigma-Aldrich], strontium(II) nitrate [Sr(NO 3 ) 2 , AR, Guangdong chemical reagent)], citric acid monohydrate (AR, LookChem.) were utilized as precursors. Preparation of SI Catalyst Solution A was prepared by dissolving Sr(NO 3 ) 2 (280 mg) and citric acid (840 mg) in 5.0 mL of deionized water. Solution B was prepared by dissolving K 2 IrCl 6 (80 mg) in 4.0 mL of ethylene glycol. Solution A was then added dropwise with stirring to solution B. The resulting mixture was dried at 150 °C for 12 h to obtain a brown solid product as a precursor. Subsequently, the precursor was calcined in air at 200 °C for 6 h, 300 °C for 6 h, 500 °C for 3 h, and 700 °C for 6 h with a heating rate of 2 °C/min. Afterward, the excess SrCO 3 impurities were removed by reacting with a 1.0 M HCl solution for 12 h to obtain SrIrO 3 (SI) catalyst. Preparation of SI 1 C 1 catalyst Solution A was prepared by dissolving Sr(NO 3 ) 2 (280 mg) and citric acid (840 mg) in 5.0 mL of deionized water. Solution B was prepared by dissolving K 2 IrCl 6 (40 mg) and Co(NO 3 ) 2 (24 mg) in 4.0 mL of ethylene glycol. The subsequent steps were identical to the preparation of the SI catalyst described above. Preparation of SI 2 C 1 catalyst Solution A was prepared by dissolving Sr(NO 3 ) 2 (280 mg) and citric acid (840 mg) in 5.0 mL of deionized water. Solution B was prepared by dissolving K 2 IrCl 6 (53 mg) and Co(NO 3 ) 2 (16 mg) in 4.0 mL of ethylene glycol. The subsequent steps were identical to the preparation of the SI catalyst described above. Preparation of SI 4 C 1 catalyst Solution A was prepared by dissolving Sr(NO 3 ) 2 (280 mg) and citric acid (840 mg) in 5.0 mL of deionized water. Solution B was prepared by dissolving K 2 IrCl 6 (64 mg) and Co(NO 3 ) 2 (10 mg) in 4.0 mL of ethylene glycol. The subsequent steps were identical to the preparation of the SI catalyst described above. Preparation of SI 6 C 1 catalyst Solution A was prepared by dissolving Sr(NO 3 ) 2 (280 mg) and citric acid (840 mg) in 5.0 mL of deionized water. Solution B was prepared by dissolving K 2 IrCl 6 (68 mg) and Co(NO 3 ) 2 (7 mg) in 4.0 mL of ethylene glycol. The subsequent steps were identical to the preparation of the SI catalyst described above. Preparation of SI 8 C 1 catalyst Solution A was prepared by dissolving Sr(NO 3 ) 2 (280 mg) and citric acid (840 mg) in 5.0 mL of deionized water. Solution B was prepared by dissolving K 2 IrCl 6 (71 mg) and Co(NO 3 ) 2 (5 mg) in 4.0 mL of ethylene glycol. The subsequent steps were identical to the preparation of the SI catalyst described above. Materials characterizations Characterization of the atomic-level crystal structure was performed using an aberration-corrected scanning transmission electron microscope (JEM-ARM200P, JAPAN) operated at 300 kV. Energy-dispersive X-ray (EDX) analysis was used to measure the relative elemental content. X-ray diffraction (XRD) patterns of SrIrO 3 were recorded on an X-ray diffractometer (Smart lab) using Cu-Kα radiation ( λ = 1.5418 Å) with a step size of 0.02° and a step time of 0.2 s in the 20°–80° range. X-ray photoelectron spectroscopy (XPS) was performed using a Thermo Scientific K-Alpha X-ray photoelectron spectrometer, and all XPS spectra were calibrated using the C 1 s line at 284.8 eV. The surface morphology of SrIrO 3 was characterized using a scanning electron microscope (TESCAN MIRA LMS). Considering the high acid resistance of SrIrO 3 , anti aqua regia was prepared by mixing hydrochloric acid and nitric acid in a 1:3 ratio for the experiment. In this solution, 1.0 mg of SrIrO 3 powder was dissolved in 10 mL of aqua regia and left to stand for 1–3 week after thorough ultrasonic treatment. Finally, the proportions of each element in SrIrO 3 were determined by ICP-MS (iCAP RQ) analysis. In situ characterizations and LOER confirmation X-ray absorption spectra of Ir L -edge were obtained at the BL17B and BL20U1 beamline of the Shanghai Synchrotron Radiation Facility (SSRF). The spectra were collected either in transmission mode or fluorescence mode using a Lytle detector. The corresponding reference samples were collected in transmission mode. The samples were ground and uniformly applied to special adhesive tape. In situ XANES characterizations were performed in fluorescence mode at the same beamline. The samples were sprayed onto carbon paper at a loading of 1.0 mg cm −2 as the working electrode. The measurements were conducted under the same conditions as the OER measurements in a self-designed cell. The in situ Raman spectroscopy characterizations were carried out using an inVia confocal Raman microscope from Renishaw. The laser power was set at 532 nm with 1% power at a grating of 1800 mm/1, the silicon peak was calibrated before testing. During the OER process, differential electrochemical mass spectrometry (DEMS) measurements were conducted using the QAS 100 apparatus from Shanghai Linglu Instruments to determine the volatile reaction products of the SI series catalysts and IrO 2 catalyst labeled with 18 O. Saturated Ag/AgCl and Pt wires served as the reference electrode (RE) and counter electrode (CE), respectively. The working electrode (WE) was prepared by sputtering Au onto a 50 μm-thick porous PTFE membrane, followed by depositing 10 μL of catalyst ink (1.0 mg/mL) onto the Au surface. The catalyst isotopic labeling was achieved by cycling the electrode in H 2 18 O for eight cycles using cyclic voltammetry (CV) with a scan rate of 5 mV/s in the range of 0–0.5 V vs. Ag/AgCl. Subsequently, the 18 O-labeled electrode was rinsed with H 2 16 O to remove residual H 2 18 O. Finally, the electrode was electrochemically tested against Ag/AgCl in a 1.0 M H 2 SO 4 solution at different potentials with a scan rate of 5 mV/s. The DEMS signal was normalized by current density (A/g). Simultaneously, real-time measurements of gas products with different molecular weights generated during the OER process were conducted using mass spectrometry. In situ ICP-MS experiments were performed using a Thermo Scientific iCAP RQ instrument. The experimental setup consisted of a standard three-electrode cell with a 3 mm glassy carbon working electrode, consistent with the electrochemical testing. The reference electrode used was a saturated calomel electrode (Hg/HgCl 2 ), and the counter electrode was a platinum foil electrode. To ensure accurate detection of ion distribution, a stirrer was employed to prevent leaching and dissolution errors, with data sampling occurring every 15 s. Electrochemical characterizations To prepare the catalyst ink, a 0.5 mg amount of catalyst was mixed with 1.0 ml of a 0.05 wt% Nafion solution and neutralized. Subsequently, a 10 μl volume of the prepared ink was deposited onto a glassy carbon electrode (GCE) with a diameter of 5 mm and dried using an infrared lamp. Prior to use, the GCE was polished with 0.05 μm alumina powder and rinsed three times with a mixture of high purity water and ethanol. Electrochemical measurements were conducted in a three-electrode system using an electrochemical workstation (CHI 760E). The reference electrode used was an Hg/HgCl 2 electrode in a 0.5 M H 2 SO 4 electrolyte, while a carbon rod served as the counter electrode. The working electrode was the GCE with the catalyst. LSV and CV was performed in 0.5 M H 2 SO 4 solution at a scan rate of 10 mV/s. A home-made PEM water electrolysis cell with a proton exchange membrane was used to evaluate the performance of SI series catalyst. The preparation step of catalyst inks is the same as above method. The total catalyst loading on the electrode was 1.0 mg and all the catalyst inks were deposited on carbon paper (1 cm × 1 cm). The cell temperature (25, 65, and 85 °C) was maintained by an electric heating plate and measured by a temperature probe in electrolyte. Computational methods Spin-polarized density functional theory (DFT) calculations were performed in the plane wave and ultrasoft pseudopotential (USPP) with Perdew-Burke-Ernzerhof (PBE) exchange functional correction as implemented in Quantum ESPRESSO [41] , [42] . An energy cutoff of 25 Ry was employed for the plane wave expansion of the electronic wavefunction. The atomic structures of the models were fully relaxed until self-consistency was achieved with a convergence criteria of 10 −6 Ry for the energy and 10 −3 Ry/Bohr for the atomic coordinates. To prevent interaction between layers, a vacuum slab of 12 Å was used to isolate the surface. For bulk geometry optimization, a 3 × 3 × 1 Monkhorst-Pack k-point set was used, while a 5 × 5 × 1 set was used for electronic structure calculations. The correction for every adsorbate and surface, with typical values of +0.35 eV, +0.05 eV, +0.35 eV for *OH, *O and *OOH respectively. To simulate the complex unsaturated IrO x structure, we start by constructing and optimizing the slab structure of the original SrIrO 3 . Then, the surface Sr atoms were removed from the SrIrO 3 slab for further optimization. According to a previous report [25] , the Ir-O coordination number on the SrIrO 3 surface is approximately 4.5, achieved by removing 4 Sr atoms and their corresponding 3 neighboring O atoms. The same procedure can be applied to the Co-doped system, where removing a Co atom also removes 2 neighboring O atoms. XAS analysis The acquired extended X-ray absorption fine structure (EXAFS) data were processed following standard procedures using the ATHENA module of the Demeter software package [43] . 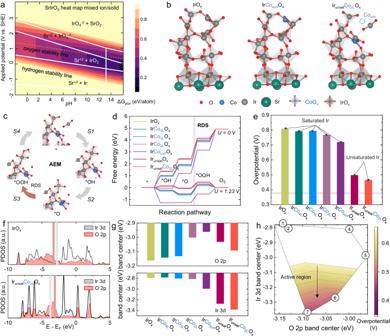Fig. 3: Theoretical calculations of SrIrO3-based perovskite catalysts. aPourbaix diagram of SrIrO3.bPossible computational models of IrOx, IrCosurfOx(surface Co doping) and IrunsatCo2LOx(second layer Co doping with unsaturated IrOx) for DFT calculations.cAdsorbate evolution mechanism (AEM) diagram.dOER free energy diagrams of different models.eOverpotential of different computational models.fDensity of states diagrams for IrOxand IrunsatCo2LOx, and (g,h) energy band center and volcano plot for different computational models. The EXAFS spectra were obtained by subtracting the post-edge background from the overall absorption and then normalized with respect to the edge-jump step. 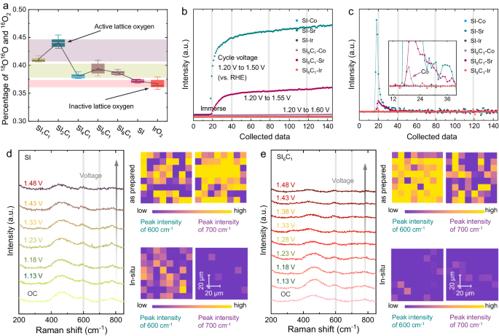Fig. 4: In situ characterizations of samples. aThe18O16O percentage of the samples test by DEMS.bIn situ ICP-MS diagram of SI and SI6C1and (c) its differential transformation diagram, in set: enlarged diagram.d,eIn situ Raman and Raman mapping of SI samples and SI6C1samples. The χ(k) data were Fourier transformed to real (R) space using a Hanning window (dk = 1.0 Å −1 ) to separate the contributions from different coordination shells. 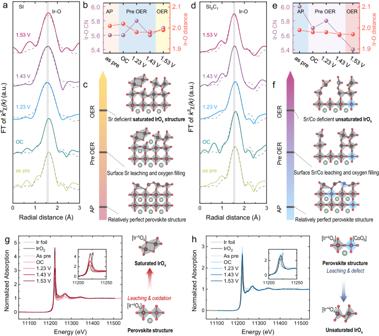Fig. 5: In situ XAS characterization of samples. aR-space fitting diagram for SI sample.bChanges in Ir-O coordination and Ir-O bond length of SI sample.cStructure change diagram of SI sample;dR-space fitting diagram of SI6C1sample.eIr-O coordination and Ir-O bond length variation diagram of SI6C1sample.fStructure change diagram of SI6C1sample.gIr–LIIIAbsorption edge diagram of SI sample, in set: enlarged diagram.hIr–LIIIabsorption edge diagram of SI6C1sample, in set: enlarged diagram. 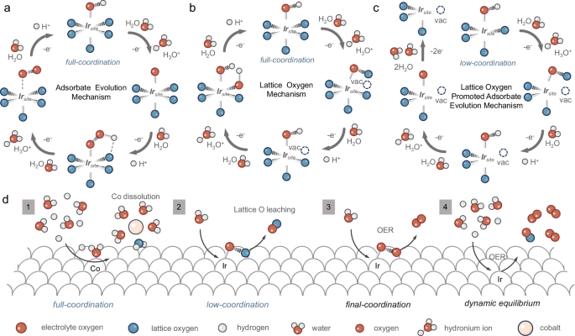Fig. 6: Proposed possible OER mechanism. aAdsorbate evolution mechanism.bLattice oxygen mechanism.cLattice oxygen promoted adsorbate evolution mechanism.dCatalytic mechanism of Co-doped SrIrO3catalyst. To determine the quantitative structural parameters around the central atoms, least-squares curve parameter fitting was performed using the ARTEMIS module of the Demeter software package.